Interface engineering of quantum Hall effects in digital transition metal oxide heterostructures Topological insulators are characterized by a non-trivial band topology driven by the spin-orbit coupling. To fully explore the fundamental science and application of topological insulators, material realization is indispensable. Here we predict, based on tight-binding modelling and first-principles calculations, that bilayers of perovskite-type transition-metal oxides grown along the [111] crystallographic axis are potential candidates for two-dimensional topological insulators. The topological band structure of these materials can be fine-tuned by changing dopant ions, substrates and external gate voltages. We predict that LaAuO 3 bilayers have a topologically non-trivial energy gap of about 0.15 eV, which is sufficiently large to realize the quantum spin Hall effect at room temperature. Intriguing phenomena, such as fractional quantum Hall effect, associated with the nearly flat topologically non-trivial bands found in e g systems are also discussed. Since the discovery [1] , [2] of the quantum Hall effect (QHE), the quest for topologically ordered states of matter has become a major subject of interest in condensed matter physics. Haldane [3] first proposed that electrons hopping on a honeycomb lattice could realize the QHE in the absence of Landau levels, pointing out the possibility of non-trivial topology in simple band insulators. Along this direction, recent efforts have culminated in the theoretical prediction [4] , [5] , [6] , [7] and subsequent experimental realization [8] , [9] , [10] of the so-called topological insulators (TIs) in materials with strong spin-orbit coupling (SOC). Many interesting phenomena, including giant magneto-electric effects [11] and the appearance of Majorana fermions [12] , have been predicted. Once realized in real materials, these phenomena could lead to entirely new device paradigms for spintronics and quantum computing. However, so far, the material realization of TIs has been limited to narrow band-gap semiconductors based on Hg or Bi, in which the electronic properties are dominated by s and p orbitals. Here, we report our theoretical investigation of topological insulating behaviour in a completely different materials class—heterostructures of transition-metal oxides (TMOs) involving d electrons. Our motivation is twofold. First, artificial heterostructures of TMOs are becoming available owing to the recent development [13] , [14] , [15] in the fields of oxide superlattices and oxide electronics [16] . In particular, layered structures of TMOs can be now prepared with atomic precision, thus offering a high degree of control over important material properties, such as lattice constant, carrier concentration, SOC and correlation strength. As we show below, these advantages can be readily exploited in the design of TIs. Second, TMOs constitute a wide class of compounds that exhibit a variety of intriguing properties and electronic states associated with the electron–electron interactions, encompassing superconductivity, magnetism, ferroelectricity and Mott insulators. Combined with the TI phase, TMO heterostructures provide a very promising platform to explore various topological effects. Our main results are summarized below. We first demonstrate the design principle for realizing two-dimensional (2D) TIs in bilayers of perovskite-type TMOs grown along the [111] crystallographic axis by using phenomenological tight-binding (TB) modelling. Based on this design principle and first-principles calculations, a number of candidate materials are identified. The topological band structure of these materials can be fine-tuned by changing dopant ions, substrates and external gate voltages, which will enable also the control of the topological quantum phase transition. In particular, we predict that LaAuO 3 bilayer has a topologically non-trivial energy gap about 0.15 eV, which is sufficiently large to realize the quantum spin Hall effect at room temperature. When electron–electron interaction is included, our system with topologically non-trivial band structure could have far more interesting physics. Here, we demonstrate this possibility by focusing on the TMO bilayers of e g systems, which are characterized by nearly flat topologically non-trivial Z 2 bands. We argue that when these bands are partially filled, electron correlation could give rise to the quantum anomalous Hall (QAH) effect and the fractional QHE. Our results may open new directions focusing on topological phenomena in the rapidly growing field of oxide electronics. Design principle To demonstrate the design principle for engineering TIs in TMO heterostructures, we consider perovskite-type TMOs as our prototype system. These compounds are very common and have the chemical formula AB O 3 , where O is oxygen and B is a transition-metal (TM) ion. The key idea is to start with a band structure that possesses 'Dirac points' in the Brillouin zone without the SOC, and then examine whether an energy gap can be opened at those points with the SOC turned on. If an energy gap does open, combined with proper filling the resulting state could be a TI. In an ideal perovskite structure, the TM ions sit on a simple cubic lattice, with the octahedral crystalline field splitting the TM d orbitals into twofold degenerate and threefold degenerate levels, well separated by so-called 10 Dq on the order of 3 eV. Such a lattice geometry usually does not support Dirac points. Instead, we consider bilayers of the perovskite structure grown in the [111] direction. 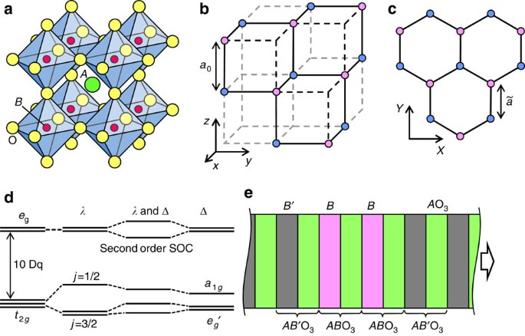Figure 1: Formation of the honeycomb lattice in a (111) bilayer in the cubic lattice. (a) Perovskite structureABO3. (b) A (111) bilayer consisting of the top layer indicated by red circles and the bottom layer indicated by blue circles. The lattice constant isa0. The bilayer shown as solid lines in (b) forms the honeycomb lattice when projected on the [111] plane with the lattice constant(c). The real space coordinates are labelled by (x,y,z) in the original cubic lattice, while it is labelled by (X,Y) in the [111] plane. (d) Level structure of TMdorbital. In the cubic environment,dorbitals split intoegandt2gmanifolds. With the SOC,t2gmanifold further splits into two levels characterized by the effective total angular momentumj=1/2 and 3/2. With the trigonal crystal field,t2gmanifold splits into two levels denoted bya1gande′g. With both the SOC and the trigonal field,t2gmanifold splits into three levels andegmanifold splits into two levels, that is, all the degeneracies are lifted except the Kramers doublets. (e)ABO3monolayer is grown onAO3-terminatedAB′O3substrate capped byAB′O3. The direction of crystal growth is indicated by an arrow. As shown in Figure 1 , the TM ions in the (111) bilayer are located on a honeycomb lattice consisting of two trigonal sublattices on different layers. This lattice geometry has three consequences: firstly, it is well known from the study of graphene that electrons hopping on a honeycomb lattice generally give rise to Dirac points in the band structure; secondly, a layer potential difference can be easily created by applying a perpendicular electric field or by sandwiching the bilayer between two different substrates, which allows experimental control of the band topology; and, thirdly, the honeycomb lattice further reduces the symmetry of the crystalline field from octahedral ( O h ) to trigonal ( C 3 v ), and introduces additional level splitting of the d orbitals. The last point turns out to be crucial for realizing the topologically insulating phase. Figure 1: Formation of the honeycomb lattice in a (111) bilayer in the cubic lattice. ( a ) Perovskite structure AB O 3 . ( b ) A (111) bilayer consisting of the top layer indicated by red circles and the bottom layer indicated by blue circles. The lattice constant is a 0 . The bilayer shown as solid lines in ( b ) forms the honeycomb lattice when projected on the [111] plane with the lattice constant ( c ). The real space coordinates are labelled by ( x,y,z ) in the original cubic lattice, while it is labelled by ( X,Y ) in the [111] plane. ( d ) Level structure of TM d orbital. In the cubic environment, d orbitals split into e g and t 2 g manifolds. With the SOC, t 2 g manifold further splits into two levels characterized by the effective total angular momentum j =1/2 and 3/2. With the trigonal crystal field, t 2 g manifold splits into two levels denoted by a 1 g and e ′ g . With both the SOC and the trigonal field, t 2 g manifold splits into three levels and e g manifold splits into two levels, that is, all the degeneracies are lifted except the Kramers doublets. ( e ) AB O 3 monolayer is grown on A O 3 -terminated AB ′O 3 substrate capped by AB ′O 3 . The direction of crystal growth is indicated by an arrow. Full size image We first consider the t 2 g manifold, in which the on-site SOC is active. In our modelling, only nearest-neighbour (NN) hopping of d electrons between the TM sites via oxygen p orbital is included. As we are interested in the band topology, which is robust against small perturbations as long as the band gap remains open, our model is justified and allows us to capture the essential ingredients with minimal parameterization. The TB Hamiltonian is given by where r and τ label the lattice sites and the t 2 g orbitals, respectively. The first term is the hopping term represented by a single amplitude t and the dimensionless structural factor . The second term is the on-site SOC, which splits the t 2 g levels into a j =1/2 doublet with energy λ and a j =3/2 quadruplet with energy − λ /2. l r and s r are the angular momentum and spin operators. The third term is the trigonal crystalline field which splits the t 2 g manifold into a 1 g and e g ′ manifolds with their level separation given by 3Δ/2. V in the last term is the layer potential difference, and ξ r = 1 when r is in the top or bottom layer. The explicit form of the Hamiltonian is presented in the Methods. The large number of orbitals (six per TM site) involved in our model give rise to a very rich behaviour of the topological band structure in the parameter space. Depending on the strength of the SOC, the system falls into two different phases. In the strong SOC limit (|λ/ t|>8/3 when Δ =0), bands originating from the j =1/2 and j =3/2 orbitals are completely separated. The trigonal crystal field then opens up an energy gap within each manifold, and a non-trivial Z 2 topology can be realized. This is similar to the results reported on Iridium compounds [17] , [18] . In the weak SOC limit, bands from j =1/2 and j =3/2 orbitals become mixed away from the Γ point. Again, we find topologically non-trivial energy gaps that can be opened by Δ. The Z 2 topological invariant is determined using two different methods. One can either evaluate it directly from the bulk band structure [19] or count the number of edge states. 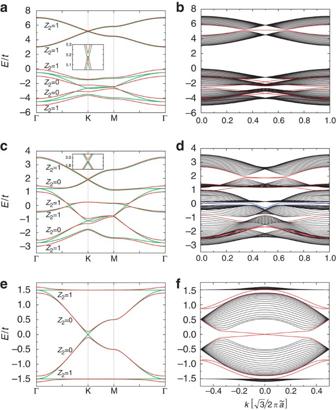Figure 2: Dispersion relations of the (111) bilayer. (a) and (b)t2gmodel in the strong SOC limit. The SOC is fixed as λ/t=5 with Δ/t=1 (red) and Δ=0 (green). (c) and (d)t2gmodel in the weak SOC limit, Δ/t=0.5 with λ/t=1.5 (red), and Δ/t=1.5 with λ/t=0 (green). (e) and (f)egmodel with(red) and(green). Figures (a), (c) and (e) show the bulk dispersion relations. The dispersions in red correspond to the topologically non-trivial bands with theZ2invariants shown for each band. Sum ofZ2in the occupied bands gives theZ2topological invariant for the corresponding filling. For example, when the lowest five bands of thet2gmodel are occupied by electrons in (a),Z2invariant becomes 1+0+0+1+1 mod 2=1. The insets in (a) and (c) show the zoom-up near the K point. Figures (b), (d) and (f) show the dispersion relations in finite-thick zigzag ribbons with the periodic boundary condition along theXdirection and the openboundary condition along theYdirection. Parameters are the same as in the bulk dispersions. Edge modes supporting the spin current are indicated by red lines. For thet2gmodel with the weak SOC, there appear four edge channels between the third and the fourth bands as shown as blue lines in consistent with theZ2number. The calculated band structure for both cases together with the Z 2 index is shown in Figure 2a–d . By inspection, we find that t 2 g 1 , t 2 g 2 , t 2 g 3 and t 2 g 5 TMOs are all possible candidates for TIs in the strong SOC limit, and t 2 g 2 , t 2 g 4 and t 2 g 5 in the weak SOC. The dependence of the band topology on the layer potential difference V is rather interesting. While increasing V will eventually destroy the Z 2 non-trivial phase, under moderate values of V , the t 2 g 3 system remains TI in the strong SOC limit, and the t 2 g 4 system in the weak SOC limit. Figure 2: Dispersion relations of the (111) bilayer. ( a ) and ( b ) t 2 g model in the strong SOC limit. The SOC is fixed as λ/ t =5 with Δ/ t =1 (red) and Δ=0 (green). ( c ) and ( d ) t 2 g model in the weak SOC limit, Δ/ t =0.5 with λ/ t =1.5 (red), and Δ/ t =1.5 with λ/ t =0 (green). ( e ) and ( f ) e g model with (red) and (green). Figures ( a ), ( c ) and ( e ) show the bulk dispersion relations. The dispersions in red correspond to the topologically non-trivial bands with the Z 2 invariants shown for each band. Sum of Z 2 in the occupied bands gives the Z 2 topological invariant for the corresponding filling. For example, when the lowest five bands of the t 2 g model are occupied by electrons in ( a ), Z 2 invariant becomes 1+0+0+1+1 mod 2=1. The insets in ( a ) and ( c ) show the zoom-up near the K point. Figures ( b ), ( d ) and ( f ) show the dispersion relations in finite-thick zigzag ribbons with the periodic boundary condition along the X direction and the openboundary condition along the Y direction. Parameters are the same as in the bulk dispersions. Edge modes supporting the spin current are indicated by red lines. For the t 2 g model with the weak SOC, there appear four edge channels between the third and the fourth bands as shown as blue lines in consistent with the Z 2 number. Full size image Next, we consider the e g manifold. It is well known that the SOC is quenched within the e g manifold so it seems that the resulting band topology should be trivial. However, similar to graphene [20] , [21] and some TM ions [22] , [23] , the SOC can still take place through the virtual excitation of electrons between e g and t 2 g levels. According to the second-order perturbation theory, the effective SOC is given by where ɛ labels the e g orbitals. Hence, the Hamiltonian can be written where the SOC magnitude is given by , with Δ E roughly being the energy difference between e g and t 2 g levels. (The explicit form of the Hamiltonian is presented in the Methods and in Supplementary Note 1 .) We find that opens up an energy gap at the Γ point and also the Dirac point located at K. From the inspection of the Z 2 topological invariant and counting the number of edge states, we found that e g 1 , e g 2 and e g 3 systems become TIs ( Fig. 2e,f ). Here, the trigonal crystalline field is also important—if all t 2 g levels are degenerated, even the second-order SOC vanishes. A layer potential difference comparable to closes the gap at the Dirac point, turning the e g 2 system into a trivial insulator. On the other hand, gaps at the Γ point are stable against this perturbation. Instead, these gaps close when the local potential difference between and is comparable to . Thus, the TI state and the Jahn–Teller effect [24] compete in real materials with the e g 1 or e g 3 configuration. Materials consideration Having established that the TIs can be realized in (111)-bilayer TMO for both t 2 g and e g configurations, we now turn to real materials. We aim to realize the integer fillings established above using TM B ions with the formal valence +3 or +4. For B 3+(4+) , we choose La (Sr) for the A -site element in both the target TMO and the insulating substrate AB ′O 3 , and Al (Ti) for the B ′-site element in the insulating substrate. Controlling the strain effects and the layer potential difference is possible by replacing A and/or B ′ with their isovalent elements. It is well known that some of the TMOs are insulating due to strong correlations [25] . Therefore, if the corresponding bulk system is heavily insulating, bilayering may not be useful. Even if the corresponding bulk system is metallic, the low dimensionality in (111) bilayers may drive the system into a Mott insulator [26] . Further, the correlation effects are expected to reduce the effective band width and increase the splitting between occupied levels and unoccupied levels. While this effect does not change the band topology in e g electron systems, this could influence the topology in t 2 g systems by modifying the crystal field splitting between a 1 g and e ′ g levels. In addition, in a system with an integer number of electrons per site, local moments could be induced by the correlation effects resulting in the magnetic ordering. If the symmetry breaking by the magnetic ordering is strong, the system could become a trivial insulator. We do not consider such complexities by focusing on rather itinerant 4 d and 5 d electrons of TM ion, yet t 2 g electron systems are more susceptible for magnetic orderings than e g electron systems because of the smaller hopping intensity. These considerations somewhat limit the choice of TM and substrate material. Our candidate materials for TIs are, therefore, LaRe 3+ O 3 as a t 2 g 4 electron system, LaRu 3+ O 3 , LaOs 3+ O 3 , SrRh 4+ O 3 and SrIr 4+ O 3 as t 2 g 5 systems, and LaAg 3+ O 3 and LaAu 3+ O 3 as e g 2 electron systems. Most of these materials have been synthesized and their references are summarized in Table 1 . LaReO 3 , LaOsO 3 and LaAgO 3 have yet to be synthesized. According to Ralle and Jansen [35] , bulk LaAuO 3 has CaF 2 structure rather than the perovskite. We expect this material shapes the perovskite structure by, for example, high-pressure synthesis and grown on a substrate with the perovskite structure. If properly synthesized, perovskite LaAuO 3 is expected to be metallic as LaAgO 3 predicted by the density functional theory (DFT) calculation [33] . We also note that growing thin films of perovskite TMOs along the [111] direction has already started [36] , [37] . While t 2 g 2 systems are also candidates for TIs, the TI state is hard to realize because of the band overlap. For e g 1 and e g 3 systems, additional effects such as longer range transfer and the Jahn–Teller effect can easily modify the dispersion relations. Table 1 List of candidate materials. Full size table We first performed the DFT calculations for the bilayers of t 2 g systems LaReO 3 , LaRuO 3 , LaOsO 3 , SrRhO 3 and SrIrO 3 (details are presented in the Methods section.) 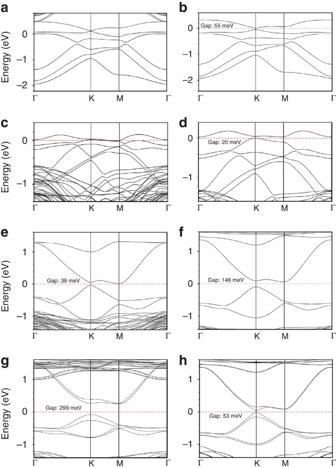Figure 3: Density functional theory results of the dispersion relations of the (111) bilayer of transition-metal oxides. Symmetric bilayers: (a) LaReO3, (b) LaOsO3, (c) SrRhO3, (d) SrIrO3, (e) LaAgO3and (f) LaAuO3. Bilayers shown in (a), (b), (e) and (f) are grown between LaAlO3, while those in (c) and (d) are grown between SrTiO3. Asymmetric bilayers of LaAuO3grown between LaAlO3and LaScO3(g), and between LaAlO3and YAlO3(h). The Fermi level is taken to be 0 of the vertical axis. Bilayers shown in (b), (d), (e), (f) and (h) are TIs with the band gap indicated, (g) is a trivial insulator and others are topological metals. Their dispersion relations are shown in Figure 3a–d . We notice the remarkable agreement between the DFT results and the TB result, Figure 2c , especially for LaReO 3 and LaOsO 3 . For SrRhO 3 , LaReO 3 and LaRuO 3 (not shown), the Fermi level crosses several bands. Thus, these systems are classified as topological metals rather than TIs. In LaOsO 3 and SrIrO 3 , the Fermi level is located inside the gap. Therefore, from the analogy to the TB model, (111) bilayers of LaOsO 3 and SrIrO 3 are TIs. From our DFT calculations, it is noted that the material dependence of the dispersion relations is rather large for t 2 g systems. This is because a large number of band parameters are involved in the band structure including the local crystalline field. Figure 3: Density functional theory results of the dispersion relations of the (111) bilayer of transition-metal oxides. Symmetric bilayers: ( a ) LaReO 3 , ( b ) LaOsO 3 , ( c ) SrRhO 3 , ( d ) SrIrO 3 , ( e ) LaAgO 3 and ( f ) LaAuO 3 . Bilayers shown in ( a ), ( b ), ( e ) and ( f ) are grown between LaAlO 3 , while those in ( c ) and ( d ) are grown between SrTiO 3 . Asymmetric bilayers of LaAuO 3 grown between LaAlO 3 and LaScO 3 ( g ), and between LaAlO 3 and YAlO 3 ( h ). The Fermi level is taken to be 0 of the vertical axis. Bilayers shown in ( b ), ( d ), ( e ), ( f ) and ( h ) are TIs with the band gap indicated, ( g ) is a trivial insulator and others are topological metals. Full size image We now move to e g 2 electron systems, LaAgO 3 and LaAuO 3 . Our DFT results for these systems are shown in Figure 3e,f . As in the t 2 g case, the DFT reproduces the TB result fairly well. In both undoped systems, the Fermi level is inside the gap at the K point, and from the analogy to the TB result, these systems are TIs. The gap amplitude is found to be about 150 meV for LaAuO 3 and 40 meV for LaAgO 3 , so these systems should remain TIs at room temperature. The band gap and topological property can be controlled by breaking the symmetry between top and bottom layers. As shown in Figure 3g , the asymmetric bilayer with LaScO 3 has larger band gap ~300 meV, and from the inspection of the symmetry of the wave function at the K point, this bilayer is a trivial insulator. On the other hand, the asymmetric bilayer with YAlO 3 has smaller band gap ~50 meV and remains to be a TI ( Fig. 3h ). Such a small band gap TI is especially useful to control the topological property by using the gate voltage. Similar to LaAgO 3 and LaAuO 3 , we also performed the DFT calculations for a 3 d system LaCuO 3 . We found that this system develops an instability towards magnetic ordering because the itinerancy is reduced compared with 4 d and 5 d systems. Nearly flat Z 2 topologically non-trivial bands One of the appealing aspect of realizing non-trivial band topology in TMOs is the rich possibilities of novel phenomena that could emerge when electron correlation is considered. Here, we demonstrate one of the possibilities in the e g systems with nearly flat Z 2 topologically non-trivial bands (see Fig. 2e ). Obviously, when the chemical potential is tuned into the nearly flat Z 2 bands, we are in a novel regime of quantum many-body physics. From the inspection of dispersion relations shown in Figure 3e and f , the upper flat band appears to be more stable than the lower flat band. Tuning the chemical potential in the upper flat band corresponds to removing electrons from d 10 systems or adding electrons to d 9 systems. When such a situation is realized, kinetic energy is suppressed and physics is controlled mainly by interaction, whose energy scale is typically 1–2 eV, much larger than the width of flat bands W ~0.2 eV. What would be the ground state of the system? Here, we propose several natural candidate states. One very likely consequence of the short-range repulsion U , when the doping of the nearly flat band is not too small, is to drive the system ferromagnetic because of Stoner's criteria U/W»1. On the other hand, when doping is too small, Wigner crystal phase should naturally occur. In the following, we assume that spontaneous ferromagnetic ordering occurs. The magnetic order should be viewed as a breaking of a discrete symmetry, due to the SOC, instead of the breaking of a continuous spin rotation symmetry, which is not realized in a 2D system at any finite temperature. Our discussion is not limited to spontaneous ordering, because magnetism can be also introduced externally by using a magnetic insulator as a substrate. 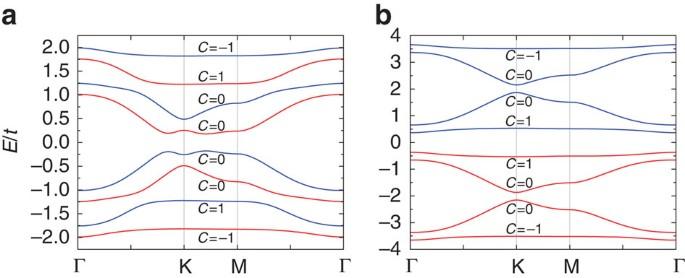Figure 4: Bulk dispersion relations of the (111) bilayer ofegmodel with the Zeeman splitting. (a) Small Zeeman splitting withB=0.3t, and (b) large Zeeman splitting withB=2t. Here, we used. Bands with the majority (minority) spin component are indicated as red (blue) lines. Band-dependent Chern number is also indicated. We model the effect of ferromagnetic ordering by adding a Zeeman spin splitting to the Hamiltonian: Resulting dispersion relations for e g system with two characteristic Zeeman fields are presented in Figure 4 . From the inspection of the Chern number, the QAH-insulating state [38] is realized in e g 0.5 and e g 3.5 systems, and also e g 1 , e g 1.5 , e g 2.5 and e g 3 systems when the Zeeman field is large. The e g 1 configuration with the large Zeeman splitting is realized in undoped perovskite manganites. More interesting physics occurs when the nearly flat 'Chern' band is partially filled (see Figs 2e and 4 ). In this case, as pointed out recently, fractional quantum Hall (FQH) states are likely to be realized [39] , [40] , [41] , [42] , [43] , [44] . To elaborate this possibility, we perform exact diagonalization calculation after projecting on-site repulsion and NN repulsion into the 1/3 filled highest Chern band (that is, at e g 3.5+1/6 ). Indeed, signatures of a ν =1/3 FQH state are observed (details of the exact diagonalization and the numerical result are presented in the Supplementary Note 2 ). We find that, when the NN repulsive interaction is larger than the width of the flat band, the ground state degeneracy is threefold on a torus, and the Chern number (excluding the integer Chern number from the filled bands) of the ground state wave function is ~1/3 up to finite size correction. Figure 4: Bulk dispersion relations of the (111) bilayer of e g model with the Zeeman splitting. ( a ) Small Zeeman splitting with B =0.3 t , and ( b ) large Zeeman splitting with B =2 t . Here, we used . Bands with the majority (minority) spin component are indicated as red (blue) lines. Band-dependent Chern number is also indicated. Full size image The aforementioned FQH effects and QAH effects are both high-temperature effects and fundamentally different from the quantum Hall states realized in GaAs 2D electron gas in a magnetic field, where quasi-particle energy gap is controlled by the long-range Coulomb repulsion (ɛ is the dielectric constant and l B is the magnetic length), typically around a few Kelvin. In the present systems, quasi-particle energy gap is determined by the short-range repulsion ~1–2 eV. This indicates that room temperature FQH effects may be realized. FQH states, in particular the non-Abelian states, have been shown to be very useful as building blocks of a quantum computer [45] , [46] . A high-temperature non-Abelian quantum Hall states in the TMO heterostructures, for example, at ν =1/2 filling where natural candidate states are in the same universality class of Pfaffian states [47] or anti-Pfaffian states [48] , [49] , if realized experimentally, would have strong impacts on both fundamental physics and its applications, including the efforts of realizing topological quantum computation. Before closing, we make few remarks on TIs in the TMO bilayers. The direct confirmation of the TI state is possible by measuring the conductance. As in Bernevig et al . [5] and König et al . [8] , the conductance should be quantized as σ =2 e 2 / h per (111) bilayer in the two-terminal measurement. The conductance can be controlled by using the gate voltage. In our DFT calculations, the (111) bilayers are repeated along the [111] axis. With the non-zero inter-bilayer coupling, the helical edge channels on the surface of the sample will turn to the two Dirac fermions at k [111] =0 and 1/2 in the unit of the reciprocal lattice vector along the [111] direction. Thus, strictly speaking, the TI is classified as a 'weak' TI and the backward scattering between the two Dirac fermions, if it exists, causes the localization. In order to avoid this, one needs to make the single (111) bilayer or keep the neighbouring (111) bilayers far apart so that the inter-bilayer coupling becomes exponentially small. When fabricating the (111) bilayer, a small number of defects would have minor effects because the edge modes surrounding them are disconnected. However, as the defect density increases, two surfaces are eventually connected through the edge modes belonging to the islands. As a result, the backward scattering takes place. Another source of the localization is islands of thicker (111) TMO layers. The suppressed trigonal field inside such thick islands is expected to create the gapless bulk modes. In further thicker islands of (111) TMO layers, metallic state would be realized inside the sample. In addition to (111) bilayers, we have studied model (111) trilayers and found that the TI states are robust without the even–odd oscillation between TI and trivial insulator, as predicted for the bismuth thin films [50] . Structurally, a (111) trilayer forms a so-called dice lattice, which could also bring about interesting quantum effects characterized by the Chern number C =±2 (ref. 51 ). Of course, if the layer structure is too thick then the bulk cubic symmetry is restored and the system is no longer a TI. So far, we did not mention the correlation effects and competing ground states except for the previous section. For limiting cases, we have performed unrestricted Hartree–Fock calculations for multi-orbital Hubbard models defined on (111) bilayers. We found that the TI states are rather robust for e g 2 systems and become unstable against antiferromagnetic insulating states when the interaction strength is comparable to the full bandwidth as in the 2D Hubbard model on the honeycomb lattice [52] . For e g 1 or e g 3 systems, the QAH-insulating states could be generated dynamically by correlation effects without the SOC [53] , [54] , yet trivial-insulating states due to the Jahn–Teller effect would also be stabilized depending on the relative balance between the Coulomb interaction and the Jahn–Teller coupling. In this paper, we focused on the perovskite-type TMOs. Thus, our design principle for the TI state works only for the [111] plane because other planes such as [001] and [110] do not support a honeycomb lattice. However, this approach is not limited to the perovskite systems. For example, the [0001] plane of corundum Al 2 O 3 , that is, sapphire, involves a honeycomb lattice formed by Al atoms. Such a system could also be utilized as the substrate material to artificially create the TI state. TB models in the real space First, we consider a general multiband TB model on a cubic lattice given by where r labels the TM sites, σ spin and μ orbitals. is a transfer matrix, which depends on the pair of orbitals but not on the spin; its detail will be presented shortly. For t 2 g electron systems, the trigonal crystal field directly couples with the local t 2 g level. In addition, the angular momentum is not quenched, and therefore the SOC is active. Including these two effects, a TB model for t 2 g systems is written as with H SO and H tri given by the second and the third terms of equation (1), respectively. The explicit form of H SO for the t 2 g -alone model is given by with the use of the following convention for the orbital index: , and . σ τ with τ = a,b,c is the Pauli matrix, and is the Levi–Civita antisymmetric tensor. The dependence of transfer matrices on the orbital and direction is given by the Slater–Koster formula [55] as follows: for the NN hopping and for the second-neighbour (SN) hopping. Here, are the unit vector along the x, y and z direction, respectively. Although it is via weak π hybridization t pd π between a TM ion and an oxygen ion, the NN hopping is the largest parameter in this model, thus, taken as the unit of energy t . Δ pd is the level difference between TM d orbitals and oxygen p orbitals. The ratio between and t π is the dimensionless parameter t δ ′ is also the NN hopping, but it is via weak direct overlap and, therefore, is expected to be small. t σ ′′ and t π ′ are the SN hoppings due to the higher-order processes involving the transfer between two oxygen ions as As involves relatively strong (weak) σ ( π ) hybridization between two oxygen ions we expect Typical transfer intensities are shown in Supplementary Fig. S1(a) . For e g electron systems, linear coupling with the trigonal crystal field is absent. Therefore, the C 3 lattice symmetry of a (111) bilayer does not influence the on-site e g level. On the other hand, e g degeneracy can be lifted by the distortion of an O 6 cage surrounding a TM ion, that is, the Jahn–Teller effect. Focusing on the metallic regime, we neglect this effect. The angular momentum is quenched unless the coupling between e g and t 2 g orbitals are considered. We also neglect this effect at the moment but reconsider it later. Thus, for the e g -alone model, The dependence of transfer matrices on the orbital and direction is again given by the Slater–Koster formula [55] . For the NN hopping, we have and for the SN hopping Here, ɛ (= α, β ) labels the e g orbitals as and For e g electron systems, the NN hopping is via strong σ hybridization between a TM ion and an oxygen ion t pd σ and, therefore, largest. This hopping integral is taken as the unit of energy t . Again, the dimensionless parameter is defined by the ratio between and t σ as The NN hopping t δ is due mainly to the direct overlap between two TM ions and, therefore, expected to be small as t δ′ in the t 2 g orbital model. t σ ′ is the SN hopping due to the higher-order processes involving the transfer between two oxygen ions as . Typical transfer intensities are shown in Supplementary Fig. S1(b) . TB models on the (111) bilayer By constraining the atomic coordinate r within the (111) bilayer R =( X,Y ), it is straightforward to derive the TB Hamiltonian as a function of 2D momentum k =( k x , k y ). We use the convention in which the projection of the NN bond into the (111) plane is taken as the unit of the length scale. This is a factor smaller than the lattice constant of the cubic perovskite, and the size of the new unit cell is Taking the primitive lattice vectors as and the first Brillouin zone is a hexagon with six corners located at For the t 2 g orbital model, we obtain with Here, the spin indices are suppressed for simplicity. ∓ V /2 is the sublattice-dependent potential, which breaks the symmetry between the top (labelled 1) and bottom (labelled 2) layers. For the e g orbital model, we obtain with DFT calculations DFT calculations were carried out using the projector augmented wave method [56] with the generalized gradient approximation in the parametrization of Perdew, Burke and Enzerhof [57] for exchange correlation as implemented in the Vienna Ab Initio Simulation Package [58] . The default plane-wave energy cutoff for O, 400.0 eV, was consistently used in all the calculations. The optimized crystal parameter is 3.81 Å for bulk LaAlO 3 , and 3.95 Å for bulk SrTiO 3 . These values are in consistent with the experimental values of 3.79 Å (Berkstresser et al . [59] ) and 3.91 Å (Hellwege and Hellwege [60] ). The TM bilayer structures were simulated by a supercell consisting of 12 A O 3 and 12 B layers along the [111] direction with ( A,B )=(La,Al) or (Sr,Ti) with two adjacent B layers replaced by TM ions. In the (111) plane, the supercell contains a 1×1 unit cell. A 6×6×1 special k -point mesh including the Γ point (0,0,0) was used for integration over the Brillouin zone. Optimized atomic structures were achieved when forces on all the atoms were <0.01 eV/Å. How to cite this article: Xiao, D. et al . Interface engineering of quantum Hall effects in digital transition-metal oxide heterostructures. Nat. Commun. 2:596 doi: 10.1038/ncomms1602 (2011).